Giant regular polyhedra from calixarene carboxylates and uranyl Self-assembly of large multi-component systems is a common strategy for the bottom-up construction of discrete, well-defined, nanoscopic-sized cages. Icosahedral or pseudospherical viral capsids, built up from hundreds of identical proteins, constitute typical examples of the complexity attained by biological self-assembly. Chemical versions of the so-called 5 Platonic regular or 13 Archimedean semi-regular polyhedra are usually assembled combining molecular platforms with metals with commensurate coordination spheres. Here we report novel, self-assembled cages, using the conical-shaped carboxylic acid derivatives of calix[4]arene and calix[5]arene as ligands, and the uranyl cation UO 2 2+ as a metallic counterpart, which coordinates with three carboxylates at the equatorial plane, giving rise to hexagonal bipyramidal architectures. As a result, octahedral and icosahedral anionic metallocages of nanoscopic dimensions are formed with an unusually small number of components. Most self-assembled cavities and capsules are based on hydrogen bonding [1] , [2] , [3] , [4] or coordination chemistry [5] , [6] , [7] , [8] , [9] , [10] , combined with a variety of linear, curved or hollow complementary fragments to build up three-dimensional architectures, for which the size and number of components is often difficult to predict. For instance, in Fujita's M n L 2n (M=Pd 2+ , L=dipyridylthiophene or dipyridylfuran) giant nanoscopic metallocages [11] , subtle variations in the ligand (furan versus thiophene) favour either M 12 L 24 or M 24 L 48 rhombicuboctahedral Archimedean constructs. In the design of chemical versions of the simpler five Platonic solids, regular cubes or octahedra require C 4 -symmetry ligand fragments to be combined with C 3 -symmetry metal counterparts, whereas icosahedral/dodecahedral constructs require 12 (or 20) building blocks of C 5 symmetry and 20 (or 12) fragments of C 3 symmetry [8] . In this context, carboxylic acid derivatives of calix[4]arene and calix[5]arene are ligands of choice for C 4 - and C 5 -symmetry components, respectively, whereas uranyl (UO 2 2+ ) constitutes an ideal C 3 -symmetry component. Indeed, polycarboxylates have been often employed as ligands for uranyl organic frameworks (UOFs) [12] , [13] , [14] or molecular assemblies [15] , [16] , [17] due to the affinity of uranyl ions for oxygen donors and the almost inexhaustible variety of the resulting architectures. A common geometry in uranyl–carboxylate [UO 2 2+ (RCOO − ) 3 ] − complexes is a hexagonal bipyramid, in which the three R groups of the carboxylate lie in the equatorial plane, orthogonally oriented to the apical - yl uranyl oxygens (see Fig. 1a for an example with benzoate) [15] , [18] , [19] . Although coordination in OH-free calixarenes at the lower rim involving the phenol oxygens is a common coordination mode [20] , [21] , we speculated that the high symmetry and univocal formation of polyhedral cages would prevail over other modes of coordination. Indeed, hexameric self-assembled aggregates and capsules arising from calixarenes or resorcinarenes with other lanthanides and transition metals have been widely studied [22] , [23] , [24] , [25] . 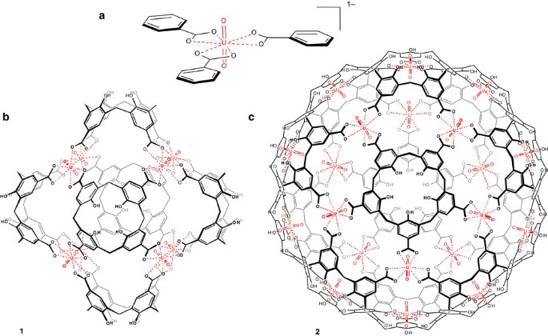Figure 1: Chemical structures of uranyl cages. (a) The hexagonal bipyramidal coordination mode of uranyl with carboxylates is illustrated for benzoic acid. (b) Chemical structure of hexameric cage1from six calix[4]arene tetracarboxylates and eight uranyl cations. (c) Chemical structure of dodecameric (icosahedral) cage2from 12 calix[5]arene pentacarboxylate fragments and 20 uranyl cations. Figure 1: Chemical structures of uranyl cages. ( a ) The hexagonal bipyramidal coordination mode of uranyl with carboxylates is illustrated for benzoic acid. ( b ) Chemical structure of hexameric cage 1 from six calix[4]arene tetracarboxylates and eight uranyl cations. ( c ) Chemical structure of dodecameric (icosahedral) cage 2 from 12 calix[5]arene pentacarboxylate fragments and 20 uranyl cations. Full size image Here we describe capsules 1 and 2 arising from calix[4]arene and calix[5]arene carboxylates and uranyl ( Fig. 1b, c ). A remarkable feature of these capsules is that the metals are not located at the corners or the edges of the resulting polyhedra, like in most of the reported examples, but on the faces instead, offering the possibility for the inner – yl oxygens to interact with guests entrapped inside the cages. Thus, the metal can act both as a gluing element for the assembly of the components and as a functional key substructure. Moreover, the resulting anionic capsules are nicely shielded structures with almost no windows, and result from an unusually small number of components and counterions, leaving a substantial amount of available inner space for host–guest interactions. All structures were fully characterised both in the solid state (X-ray diffraction) and in solution (diffusion-ordered spectroscopy (DOSY) NMR, dynamic light scattering (DLS)). Solid-state studies Tetraformylcalix[4]arene 5 was obtained as reported by Casnati at al . [26] by formylation of calix[4]arene 3 , although use of microwave heating produced quantitative yields in shorter reaction times. Although O -alkyl calix[4]arenes 9 and 10 were easily prepared by oxidation of the corresponding aldehydes by well-established procedures [27] , [28] , oxidation of 5 to the OH-free calix[4]arene 7 was only achieved by sodium chlorite [29] in a dimethylsulphoxide (DMSO)/water mixture that prevents precipitation of both the reagents and the partially oxidised intermediates. Compound 7 was isolated in good yield by simple precipitation upon addition of hydrochloric acid. Similar conditions were applied with minor modifications to calix[5]arene 4 , to obtain the unprecedented pentaformylcalix[5]arene 6 and its oxidation product 8 in good-to-moderate yields ( Fig. 2 ). 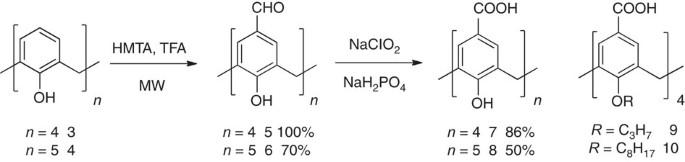Figure 2: Synthetic scheme for the preparation of calixarenes 5–10. All yields refer to purified products. Starting calixarenes3and4were obtained from the correspondingp-tert-butyl derivatives according to standard procedures. For synthetic details, seeMethods. Figure 2: Synthetic scheme for the preparation of calixarenes 5–10. All yields refer to purified products. Starting calixarenes 3 and 4 were obtained from the corresponding p - tert -butyl derivatives according to standard procedures. For synthetic details, see Methods . Full size image Formation of cages was achieved in the presence of a mild base such as pyridine, which allows deprotonation of the carboxylic acids but not of the calixarene phenol groups. In such a case, preferential coordination of the uranyl ion to the phenoxy groups would prevail, giving to the solutions a characteristic orange-reddish colour [30] , [31] , [32] . Indeed, coordination by the phenoxy groups was observed when stronger bases were employed, such as caesium or ammonium hydroxide, triethylamine or a large excess of pyridine (when used as solvent). UOFs are typically obtained by hydrothermal synthesis, a process that requires high pressures and temperatures [12] , [13] , [14] . However, for 1 and 2 , these harsh conditions only produced decomposition byproducts, whereas yellow crystals suitable for single-crystal X-ray analysis were obtained at room temperature by slow diffusion of acetonitrile on N,N -dimethylformamide (DMF) solutions of the components (calix[4]arene 7 or calix[5]arene 8 , uranyl nitrate and pyridine) at the required stoichiometries. Most remarkably, the structures of these giant supramolecular assemblies were resolved using in-house devices, a rotating anode with MoK α and two microsources with MoK α and CuK α radiation without requiring the use of a synchrotron light beam, as for many other giant assemblies [11] , [33] . The octahedral complex 1 ( Fig. 3a ) crystallises in the face-centred cubic space group Fm-3m showing a high degree of symmetry. The inner –yl oxygens of the uranyl ions define a regular hexahedron (cube) of 7.0242(15) Å edges ( Fig. 3a ). The anionic cage is made out from six calixarenes and eight uranyl subunits. The crystal packing shows that the octahedra are organised in close proximity, with an almost perfect, not interpenetrated, stacking of the aromatic walls (at 3.54 Å distance; Fig. 3c ). A top view of a two-dimensional layer ( Fig. 3d ) reveals some space between every four octahedra, with the calixarene OH groups facing the corners. Additional layers stack on top of each other, in an 'egg-box' arrangement. Likely, this space is occupied by disordered solvent molecules or counterions. 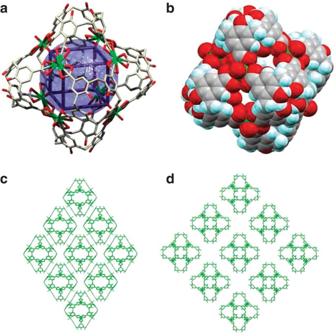Figure 3: Solid-state structure of the hexameric cage1. (a) Wireframe representation showing the cube defined by the inner−yluranyl oxygens (7.02 Å edges) and the corresponding inscribed sphere representative of an inner available volume of ca. 940 Å3. (b) Space-filling representation of the cage; (c) and (d) two views of the crystal packing along the (1 1 1) direction and theac-plane, respectively. The faces of the octahedra align in closely stacked layers (c), which display a 'eggs-box' shape when a 2D layer is seen from the top (d). Figure 3: Solid-state structure of the hexameric cage 1 . ( a ) Wireframe representation showing the cube defined by the inner −yl uranyl oxygens (7.02 Å edges) and the corresponding inscribed sphere representative of an inner available volume of ca. 940 Å 3 . ( b ) Space-filling representation of the cage; ( c ) and ( d ) two views of the crystal packing along the (1 1 1) direction and the ac -plane, respectively. The faces of the octahedra align in closely stacked layers ( c ), which display a 'eggs-box' shape when a 2D layer is seen from the top ( d ). Full size image Each capsule requires eight cationic counterions to balance the overall negative charge (one negative charge per uranyl subunit). In the crystal described in Fig. 3 , these cations are pyridines that were not localised. Thus, a polycationic counterion, such as 1,4,7,10-tetraazacyclododecane (cyclen, Fig. 4a ) that could fill the inner space, was evaluated as an encapsulated guest. Two cyclen molecules are necessary to balance the overall negative charge of each cage. Remarkably, in the resulting crystal structure, one guest molecule is located inside the cage, whereas another one fits between the corners of the hexameric aggregates ( Fig. 4b and c). The outer cyclen molecules are stabilised by hydrogen bonds with the hydroxy groups of the calixarenes. 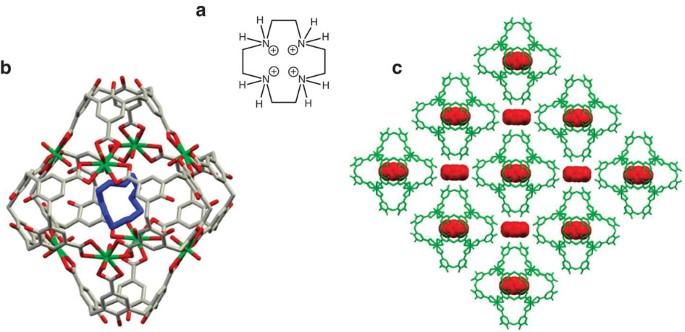Figure 4: Crystal packing of the hexameric cage 1 with cyclen. (a) Tetraprotonated 1,4,7,10-tetraazacyclododecane (cyclen). (b) Wireframe representation of the hexameric cage hosting a cyclen tetracation. (c) Crystal packing along thecaxis showing one layer of capsules with cyclen guests inside and outside the aggregates. Figure 4: Crystal packing of the hexameric cage 1 with cyclen. ( a ) Tetraprotonated 1,4,7,10-tetraazacyclododecane (cyclen). ( b ) Wireframe representation of the hexameric cage hosting a cyclen tetracation. ( c ) Crystal packing along the c axis showing one layer of capsules with cyclen guests inside and outside the aggregates. Full size image When O -alkyl calix[4]arenes 9 and 10 were employed, the corresponding octahedral crystal structures 11 and 12 , analogous to 1 , were obtained as well ( Supplementary Figs S1 and S2 ). Cage 11 spontaneously crystallised in DMF, whereas crystals of structure 12 required slow diffusion of acetonitrile on a tetrachloroethane (TCE) solution of the components. Although neither 10 nor uranyl nitrate are soluble in TCE, the mixture of both components becomes soluble after 3 days shaking in the presence of pyridine, as soon as cage 12 forms. Because of the presence of bulky O -alkyl chains at the lower rim of each calixarene, close packing of the octahedral cages was not observed. In cage 12 , bearing long O -octyl chains, the octahedron was slightly distorted. Pyridinium cations, balancing the charges of both aggregates 11 and 12 , could be located either inside or outside the cages. In 11 , three pyridinium counterions are located within the facing propyl chains and in the inner cage of the octahedron diagonal. In the case of cage 12 , bearing longer O -octyl chains, four counterions were observed in close packing inside the cage (together with a water molecule), whereas the remaining four counterions were outside. Another Platonic solid, icosahedron 2 ( Fig. 5a ), was formed when calix[5]arene pentacarboxylic acid 8 was used. In this case, 12 calixarenes displaying a wide-open cone conformation are placed at the vertices, whereas 20 uranyl ions glue the ensemble at each of the faces. Twenty additional pyridinium ions are counterbalancing the negative charges, although only two were located for each capsule, in the space available at the lower rim between two spherical aggregates. Overall, the structure is made of 32 pieces and 20 counterions, a remarkably low number of components relative to other metallocages, such as Fujita's giant cage of slightly bigger size (72 pieces + 24 PF 6 − counterions) [11] . If we approximate the cage to a sphere, this would have a diameter of 3.65 nm and an outer volume of ca. 25.5 nm 3 . 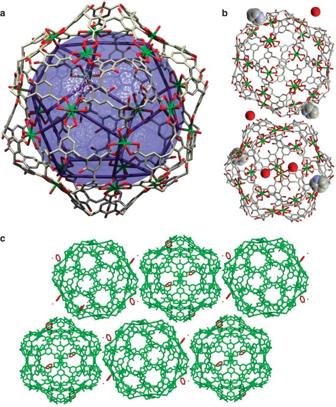Figure 5: Solid-state structure of the icosahedral cage2. (a) Wireframe representation showing aquasi-dodecahedron defined by the inner−yluranyl oxygens with edges between 8.24 and 9.07 Å, and an inscribed sphere of ca. 12 Å radius (7238 Å3volume), representative of the inner available space. (b) Position of the pyridinium counterions interacting with the oxygen of the uranyl and water molecule hydrogen bonded to an OH group of the lower rim. (c) View of the crystal packing. The cavity is likely filled with disordered pyridinium cations and solvent molecules. Figure 5: Solid-state structure of the icosahedral cage 2 . ( a ) Wireframe representation showing a quasi -dodecahedron defined by the inner −yl uranyl oxygens with edges between 8.24 and 9.07 Å, and an inscribed sphere of ca. 12 Å radius (7238 Å 3 volume), representative of the inner available space. ( b ) Position of the pyridinium counterions interacting with the oxygen of the uranyl and water molecule hydrogen bonded to an OH group of the lower rim. ( c ) View of the crystal packing. The cavity is likely filled with disordered pyridinium cations and solvent molecules. Full size image The packing is very compact without interpenetration of the capsules, although sizable holes of ca. 1,500 Å 3 total volume are present between the hydrogen-bonded spheres. This arrangement is due to hydrogen bonding between the hydroxyl groups at the lower rims and the outer − yl oxygens. Two pyridinium cations could be located hydrogen bonded to one of the outer −yl oxygens ( Fig. 5b and c ). No attempts were made to prepare conical O -alkyl derivatives of calix[5]arene 8 . Indeed, it has been reported that O -benzyl calix[5]arene displays a 1,2-alternate conformation in the solid state [34] , and longer tails, such as octyl, produce mixtures of different conformations [35] . Solution studies The formation of cages 1 , 2 , 11 and 12 was also studied in solution by NMR and DLS. 1 H and DOSY NMR spectroscopy at 300 K showed that cage formation was highly dependent on the solvent used and on the concentration of the sample. Cages 1 , 2 and 11 were analysed in DMF− d 7 , whereas spectra of 12 were taken in a 1/1 DMF− d 7 /TCE− d 2 mixture. In all cases, it was possible to distinguish the signals for the cage and the free calixarene ( Supplementary Figs S3, S5, S7 and S9 ), revealing a slow equilibrium in the NMR time scale (see Supplementary Tables S1 and S2 for apparent stability constants). For instance, the aromatic proton signal of monomeric calixarene 7 at 7.80 p.p.m. slightly shifts to 7.78 p.p.m. upon addition of uranyl nitrate, or to 7.74 p.p.m. in the presence of pyridine, as the anionic carboxylates are formed. When both components are added to the solution of monomer, the cage forms and the monomer signal stays at 7.75 p.p.m., whereas a new broad signal corresponding to the cage arises at ca. 8.38 p.p.m. ( Supplementary Fig. S3 ). DOSY spectra ( Supplementary Fig. S4 ) confirm that cage 1 is formed only when both uranyl nitrate and pyridine are present along with the calix[4]arene. This arises from the fact that only one species diffusing slower than the calixarene is present along with the ligand and the solvent. A single large species was also present in the case of calix[5]arene 8 and cage 2 , along with the monomeric calixarene ( Supplementary Figs S5 and S6 ). A mixture of both cages, formed independently, did not reveal significant changes in the DOSY spectra, both species existing independently in equilibrium ( Fig. 6 ). 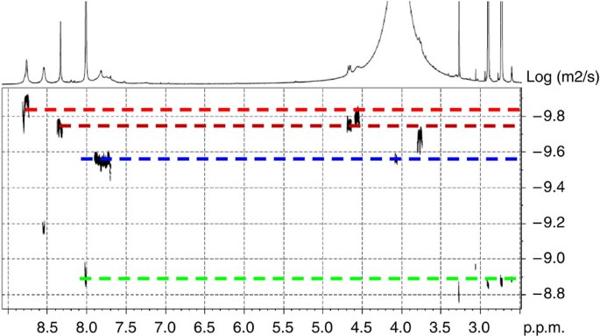Figure 6: DOSY spectrum of a mixture of cages 1 and 2 in DMF–d7at 300 K. Ligands7and8were at 6 and 12 mM concentration, respectively. DOSY NMR diffusion coefficients, calculated on the basis of monodimensional fitting and expressed in cm2s−1, are (from top to bottom in the spectrum): cage2(1.22 E-06), cage1(1.77 E-06), compounds7and8(3.10 E-06), DMF–d7((1.37±0.02) E-05). Figure 6: DOSY spectrum of a mixture of cages 1 and 2 in DMF– d 7 at 300 K. Ligands 7 and 8 were at 6 and 12 mM concentration, respectively. DOSY NMR diffusion coefficients, calculated on the basis of monodimensional fitting and expressed in cm 2 s −1 , are (from top to bottom in the spectrum): cage 2 (1.22 E-06), cage 1 (1.77 E-06), compounds 7 and 8 (3.10 E-06), DMF– d 7 ((1.37±0.02) E-05). Full size image Similarly, DOSY spectra of cages 11 ( Supplementary Fig. S8 ) and 12 ( Supplementary Fig. S10 ) show the presence of only one species with a diffusion coefficient lower than the calixarene ligand. Diffusion coefficients and hydrodynamic radii are correlated theoretically by the Stokes–Einstein equation, which requires the diffusion coefficient to be determined at infinite dilution [36] . Other factors, such as concentration, temperature, fluctuation, convection and viscosity changes are also influential [37] , [38] . In our case, these problems could not be handled by means of calibration with an internal reference, as we were unable to find suitable standards of similar sizes and shapes. For these reasons, no quantitative estimation of our cages' sizes was attempted by DOSY, and DLS was employed instead. Only one Gaussian distribution was observed for each compound in DMF, and the observed hydrodynamic radii were in full agreement with the dimensions of the cages in the solid state ( Supplementary Fig. S11 ). Thus, for OH-unsubstituted cages 1 and 2 , the measured radii were 1.226 and 1.699 nm, respectively, which nicely fit with the 1.2- and 1.7-nm values estimated from the crystal structures. For O -alkyl derivatives of the hexameric cages 11 and 12 , the radii were 1.236 and 1.472 nm, consistent with the dimensions of an octahedron but slightly smaller than the estimated radii from the solid state structures (1.6 and 2.1 nm, respectively), although it is likely that alkyl chains in the polar DMF solutions do not fully extend as in the crystal. A common feature of the UOFs is the presence of strong U=O bonds in the linear structure of the uranyl cation, which forces coordination of additional ligands at the equatorial positions, with the −yl oxygens in an almost perpendicular orientation. The lack of axial coordination favours formation of one-dimensional chains or two-dimensional sheets, but makes difficult the formation of well-organised and predictable three-dimensional structures, in particular when planar aromatic ligands are employed [12] . To the best of our knowledge, fullerene type, polyhedral cages have been described by Burns et al . [39] from uranyl peroxide components [40] , [41] , without organic moieties involved in the cage framework. However, use of bowl-shaped calixarene carboxylic acids allows assembly into defined and unique globular assemblies, built up from organic ligands and uranyl, in which the uranyl groups are centred in the faces of regular polyhedra. We have shown that calix[4]arenes promote self-assembly into hexameric cages, whereas calix[5]arene gives rise to icosahedral structures, with a remarkable economy in the number of organic ligands required for the assembly. Thus, hexameric cages with an available spherical volume of ca.940 Å 3 inside the inner −yl oxygens are obtained with six calix[4]arene fragments, whereas a dodecameric cage with an available volume of more than 7000 Å 3 results from the assembly of only 12 calix[5]arene subunits. The cavities of the calixarene subunits are oriented towards the centre of the cage, so the overall inner volume is maximised. Consequently, the lower rim of each calixarene protrudes away from the cavity, contributing to the stability of a close-packed, non-interpenetrated, hydrogen-bonded three-dimensional network in OH-free calixarenes, or to the solubility of the aggregates in organic solvents in the case of O -alkyl derivatives. The calixarene–uranyl capsules described here are anionic, in contrast to most of the so-far reported metallo-capsules. As each uranyl subunit contributes one negative charge to the overall structure, the number of counterions needed is also limited, making the cavities ideally tailored for the encapsulation of polycationic or electron-deficient guest molecules. UOFs are photoluminiscent and simultaneously exhibit interesting photocatalytic properties that can lead to efficient degradation of organic molecules, including pollutants, under UV irradiation. Moreover, photoelectrical conversion behaviour has been reported for uranyl extended structures [42] . It is likely that confinement of several uranyl moieties into well-defined, spherical structures of nanoscopic size, such as those reported here, will contribute to exploit these properties in catalysis and photoelectronics [12] , [14] . Measurements 1 H and 13 C NMR spectra were recorded on Bruker DRX-500 (500 MHz) and AV-400 (400 MHz) spectrometers. All NMR spectral data were collected at 300 K unless otherwise specified, and chemical shifts were reported as the delta scale in p.p.m. All HR Mass spectra were recorded on Maldi TOF Bruker Autoflex. DLS data were collected at 293 K by Malvern NanoZS instrument. Single-crystal X-ray diffraction data were collected on a Bruker FR591 rotating anode equipped with Montel mirrors with MoK α radiation ( λ =0.71073 Å) and a Bruker Apex-II Duo diffractometer equipped with a microsources of CuK α ( λ =1.54178 Å) and MoK α radiation ( λ =0.71073 Å), and cooled with an Oxford Cryostream low-temperature device ( T =100(2) K). See Supplementary Figs S12–S16 for ORTEP diagrams for capsules 1 , 2 , 1 with cyclen, 11 and 12 , respectively. The Cambridge Crystallographic Data Centre entries 856,283, 856,284, 856,285, 856,286 and 856,287 contain the supplementary crystallographic data for this paper. These data can be obtained free of charge via www.ccdc.cam.ac.uk/conts/retrieving.html (or from the Cambridge Crystallographic Data Centre, 12 Union Road, Cambridge CB2 1EZ, UK; fax: (+44) 1223-336-033; or e-mail: deposit@ccdc.cam.ac.uk; see Supplementary Data 1 , 2 , 3 , 4 and 5 ). Synthesis of materials Solvents and reagents were purchased from Scharlau Chemie SA, Panreac Química SAU, Acros Organics, Sigma-Aldrich Co. and Deutero GmbH. All chemicals were used without further purification. Compounds 3 [43] , 4 [44] , 9 [27] and 10 [28] were obtained according to literature procedures. Compound 5 was prepared using a modified literature procedure [26] in a microwave reactor at 110 °C for 3 h. Compound 7 was obtained by a different procedure from the one reported in the literature [45] . 5,11,17,23,29-Pentaformyl-25,26,27,28,29-pentahydroxycalix[5]arene (6) In a sealed vial (20 ml), 25,26,27,28,29-pentahydroxycalix[5]arene ( 4 ) (159 mg, 0.300 mmol) and hexamethylenetetramine (1.60 g, 11.4 mmol) were dissolved in trifluoroacetic acid (12.0 ml), and the reaction mixture was heated at 140 °C for 5 h under microwave irradiation. A volume of 35 ml of 1 M HCl and 35 ml of CHCl 3 were added to the crude mixture, and the two-phase system was stirred overnight at room temperature. The aqueous phase was extracted again with CHCl 3 , and the collected organic phases were washed once with water. The solvent was evaporated at reduced pressure, and trituration from dichloromethane afforded a dark yellow solid (140 mg, 70%); mp: >360 °C (dec.); 1 H-NMR (400 MHz, DMSO- d 6 ) δ 9.66 (s, 5H, CHO), 7.61 (s, 10H, CH), 3.84 (s, 10H, CH 2 ); 13 C-NMR (100 MHz, DMSO- d 6 ) δ 190.8 (CHO), 161.3 (C–OH), 130.6 (CH), 128.7 ( C -CH 2 ), 127.3 ( C -CHO), 31.33 (CH 2 ); HRMS (m/z): [M − ] calculated for C 40 H 29 O 10 669.1761; found, 669.1784 (see Supplementary Fig. S17 ). 25,26,27,28,29-Pentahydroxycalix[5]arene-5,11,17,23,29-pentacarboxylic acid (8) To a stirred mixture of pentaformylcalix[5]arene ( 6 ) (140 mg, 0.209 mmol) in DMSO (2.6 ml) and sodium dihydrogen phosphate (30 mg, 0.250 mmol) in 1.8 ml of water, a solution of sodium chlorite (0.264 g, 2.92 mmol) in 1.5 ml of water was added dropwise at room temperature over 3 h. The reaction was stirred overnight at room temperature, and was then acidified with concentrated HCl and kept overnight in the refrigerator. The solid formed was filtered, washed with water, then with methanol, and dried to give pure compound 8 as a brown solid (78 mg, 50%); mp: >350 °C (dec.); 1 H-NMR (400 MHz, DMSO- d 6 ): 7.66 (s, 10H, CH), 3.80 (s, 10H, CH 2 ). 13 C-NMR (100 MHz, DMSO- d 6 ): 167.8 (C quat –OH), 130.7 (CH), 128.4 ( C -CH 2 ), 121.0 ( C -COOH), 31.83 (CH 2 ). HRMS (m/z): calculated for C 40 H 29 O 15 749.1585; found, 749.1538 (see Supplementary Fig. S18 ). Octahedral cage 1 A mixture of 7 (20 mg, 0.033 mmol), uranyl nitrate hexahydrate [UO 2 (NO 3 ) 2 ·6H 2 O] (17.5 mg, 0.044 mmol) and pyridine (11 μl, 0.133 mmol) was dissolved in DMF (1 ml). Slow diffusion of acetonitrile at room temperature afforded yellow crystals suitable for X-ray analysis after 10 days. Octahedral cage 1 with 1,4,7,10-tetraazacyclododecane (cyclen) A mixture of 7 (5.0 mg, 0.008 mmol), uranyl nitrate hexahydrate [UO 2 (NO 3 ) 2 ·6H 2 O] (5.6 mg, 0.011 mmol) and pyridine (3 μl, 0.033 mmol) was dissolved in DMF (0.3 ml), and was added to a suspension of cyclen (2 mg, 0.012 mmol) in 0.2 ml of DMF. The mixture was shacked for a day until complete dissolution. Slow diffusion of acetonitrile at room temperature afforded yellow crystals suitable for X-ray analysis after 10 days. Octahedral cage 11 A mixture of 9 (9.7 mg, 0.013 mmol) and uranyl nitrate hexahydrate (8.6 mg, 0.017 mmol) was dissolved in DMF- d 7 (470 μl) and pyridine- d 5 (4 μl, 0.050 mmol) was added. After 1 week, yellow crystals suitable for X-ray analysis were formed. Octahedral cage 12 A mixture of tetra- O -octylcalix[4]arene tetracarboxylic acid 10 (10 mg, 0.010 mmol), uranyl nitrate hexahydrate [UO 2 (NO 3 ) 2 ·6H 2 O] (7.0 mg, 0.014 mmol) and pyridine (4 μl, 0.042 mmol) was dissolved in 1,1,2,2-TCE (0.4 ml), and the mixture was shaken for 3 days until complete dissolution. Slow diffusion of acetonitrile at room temperature afforded yellow crystals suitable for X-ray analysis after 10 days. Icosahedral cage 2 A mixture of 8 (16 mg, 0.021 mmol), uranyl nitrate hexahydrate [UO 2 (NO 3 ) 2 ·6H 2 O] (15 mg, 0.038 mmol) and pyridine (9 μl, 0.107 mmol) was dissolved in DMF (0.7 ml). Slow diffusion of acetonitrile at room temperature afforded yellow crystals suitable for X-ray analysis after 10 days. How to cite this article: Pasquale, S. et al . Giant regular polyhedra from calixarene carboxylates and uranyl. Nat. Commun . 3:785 doi: 10.1038/ncomms1793 (2012).